Modification of DBC1 by SUMO2/3 is crucial for p53-mediated apoptosis in response to DNA damage DBC1 is a major inhibitor of SIRT1, which plays critical roles in the control of diverse cellular processes, including stress response and energy metabolism. Therefore, the DBC1–SIRT1 interaction should finely be regulated. Here we report that DBC1 modification by Small Ubiquitin-like Modifier 2/3 (SUMO 2/3), but not by SUMO1, is crucial for p53 transactivation under genotoxic stress. Whereas etoposide treatment reduced the interaction of DBC1 with SENP1, it promoted that with PIAS3, resulting in an increase in DBC1 sumoylation. Remarkably, the switching from SENP1 to PIAS3 for DBC1 binding was achieved by ATM/ATR-mediated phosphorylation of DBC1. Furthermore, DBC1 sumoylation caused an increase in the DBC1–SIRT1 interaction, leading to the release of p53 from SIRT1 for transcriptional activation. Consistently, SENP1 knockdown promoted etoposide-induced apoptosis, whereas knockdown of PIAS3 or SUMO2/3 and overexpression of sumoylation-deficient DBC1 mutant inhibited it. These results establish the role of DBC1 sumoylation in the promotion of p53-mediated apoptosis in response to genotoxic stress. SIRT1, a mammalian orthologue of yeast silent information regulator 2 (Sir2), is a NAD + -dependent deacetylase [1] . SIRT1 deacetylates a variety of cellular proteins, including histones, p53, PGC1α, forkhead transcription factors, NFκB, Ku70, MyoD and PPARγ, implicating its important roles in the control of diverse cellular processes, such as gene silencing, stress response, DNA repair, heterochromatin formation, and fat and glucose metabolism [2] , [3] , [4] , [5] , [6] , [7] , [8] . In addition, SIRT1 was shown to extend the lifespan of yeast, C. elegans , and Drosophila [9] , [10] , [11] , although this effect depends on the genetic background of the organisms [12] . Given the important physiological functions, the activity of SIRT1 is regulated by multiple mechanisms, including the cellular NAD + level [13] , the endogenous inhibitor nicotinamide [14] , and post-translational modifications, such as phosphorylation and sumoylation [15] , [16] , [17] . In addition, active regulator of SIRT1 (AROS) was shown to activate SIRT1 through protein–protein interaction [18] . DBC1 was initially identified as a putative tumour suppressor, since its gene was found in a region frequently deleted in breast cancers [19] . Intriguingly, DBC1 was later found to be a negative regulator of SIRT1 (refs 19 , 20 ). DBC1-mediated inhibition of SIRT1 leads to an increase in p53 acetylation and thereby the p53-mediated processes, such as apoptosis. On the other hand, downregulation of DBC1 results in SIRT1-mediated p53 deacetylation and inhibition of stress-induced apoptosis. Moreover, by using DBC1 knockout mice, DBC1 was shown to act as a major regulator of SIRT1 in vivo [21] . DBC1 inhibits SIRT1 by direct binding to its deacetylase core and disrupting its interaction with substrates [19] , [20] . Recently, a C-terminal region that is essential for SIRT1 activity (called ESA) was shown to interact with the catalytic core [22] . Therefore, it was proposed that DBC1 competes with the ESA region for interacting with the deacetylase core, leading to inhibition of SIRT1. DBC1 may also regulate SIRT1 activity by sensing NAD + through its catalytically inactive Nudix hydrolase (MutT) domain, which is known to bind NAD + and ADP-ribose [23] . The interaction between SIRT1 and DBC1 appears to be dynamically regulated. Starvation leads to a decrease in the SIRT1–DBC1 interaction, resulting in an increase in SIRT1 activity in the liver of mice, and this effect on SIRT1 activity can be revered upon feeding with high-fat diet [21] . Interestingly, activation of cAMP/PKA pathway causes dissociation of the SIRT1–DBC1 complex in an AMPK-dependent manner, suggesting that AMPK-mediated phosphorylation of SIRT1, DBC1 or both may negatively regulate their binding [24] . Conversely, ATM/ATR-mediated phosphorylation of DBC1 increases its interaction with SIRT1 in response to genotoxic stress, leading to promotion of p53 acetylation and cell death [25] , [26] . Small Ubiquitin-like Modifier (SUMO) is an ubiquitin-like protein that is conjugated to a variety of cellular proteins. Like ubiquitin, SUMO is conjugated to target proteins by a three-step enzyme system: E1 activating enzyme (SAE1/SAE2), E2 conjugating enzyme (Ubc9) and E3 ligases (PIASs) [27] , [28] , [29] . Conjugated SUMO can be removed by a family of SUMO-specific proteases (SENPs) [30] , [31] . This reversible sumoylation process participates in the control of various cellular processes including transcription, nuclear transport and signal transduction [32] , [33] , [34] , [35] , [36] . Moreover, sumoylation has been implicated in the control of DNA damage response [37] , [38] , [39] , [40] , [41] , [42] , [43] , [44] , [45] . For example, hnRNP-K, a coactivator of p53, is sumoylated in response to DNA damage and this modification leads to hnRNP-K stabilization and p53-mediated cell cycle arrest [46] , [47] . In the present study, we demonstrated that genotoxic stress induces the modification of DBC1 at Lys591 by SUMO2/3, but not by SUMO1. We also identified PIAS3 as a DBC1-specific SUMO E3 ligase and SENP1 as a desumoylating enzyme for DBC1. Etoposide treatment markedly decreased the interaction of DBC1 with SENP1, whereas it promoted that with PIAS3. Remarkably, the switching of the binding partners of DBC1 was achieved by ATM/ATR-mediated phosphorylation of DBC1. Moreover, DBC1 sumoylation caused a dramatic increase in the DBC1–SIRT1 interaction, which led to the release of p53 from SIRT1 for transcriptional activation. Knockdown of SENP1 promoted etoposide-induced apoptosis, whereas that of SUMO2/3 or PIAS3 and overexpression of sumoylation-deficient DBC1 mutant inhibited it. These results indicate that DBC1 sumoylation plays a crucial role in the control of p53-mediated apoptosis under DNA damage conditions. DBC1 is a target for sumoylation The consensus sequence for sumoylation is Ψ-Lys-X-Glu/Asp, where Ψ is a large hydrophobic amino acid and X is any amino acid [33] . Upon sequence analysis, human DBC1 was found to have three potential sumoylation sites: Lys591, Lys667 and Lys839 ( Fig. 1a ). Therefore, we first examined whether DBC1 can be sumoylated upon overexpression of three SUMO isoforms. Interestingly, DBC1 was modified by SUMO2 and SUMO3, but not by SUMO1 ( Fig. 1b ). To identify the SUMO acceptor site(s) in DBC1, each of the Lys residues was substituted by Arg. The K591R mutation, but not the others, completely prevented DBC1 sumoylation ( Fig. 1c ), indicating that Lys591 serves as the major SUMO acceptor site. Since SUMO2 and SUMO3 show >95% identity in their amino acid sequences, we used short hairpin RNAs (shRNAs) directed to their identical nucleotide sequence for knocking down both of them, but used only SUMO3 for overexpression. 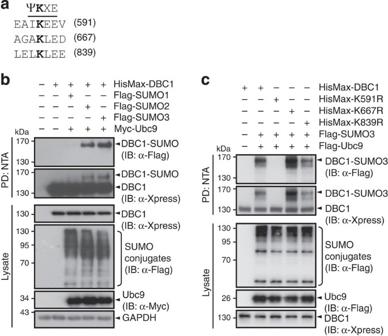Figure 1: DBC1 is a target for sumoylation. (a) Three candidate sites for sumoylation in DBC1 are shown in bold. (b) Flag-tagged SUMO isoforms were expressed in HEK293T cells with HisMax-DBC1 and Myc-Ubc9. Cell lysates were subjected to pull-down (PD) with NTA-resins followed by immunoblot analysis. The lysates were also directly probed with the indicated antibodies. (c) HisMax-tagged DBC1 and its K-to-R mutants were expressed in HEK293T cells with Flag-SUMO3 and Flag-Ubc9. Cell lysates were treated as inb. In parenthesis, the antibody used for immunoblot analysis of each gel panel was indicated. If not shown, the antibody used was generated directly to the protein indicated by the arrowhead. Note that the membrane blots obtained from immunoprecipitation were typically exposed to X-ray films for about 30 s to show up sumoylated DBC1 bands, while those obtained from cell lysates were for about 2–3 s to show just DBC1 bands for their equal expression. However, sumoylated bands could also be seen in the blots from cell lysates if exposed for a longer period (~30 s). An example is shown in the bottom panel ofbfull blots inSupplementary Fig. 12. (See also the bottom panel ofFig. 2afull blots as an additional example). Figure 1: DBC1 is a target for sumoylation. ( a ) Three candidate sites for sumoylation in DBC1 are shown in bold. ( b ) Flag-tagged SUMO isoforms were expressed in HEK293T cells with HisMax-DBC1 and Myc-Ubc9. Cell lysates were subjected to pull-down (PD) with NTA-resins followed by immunoblot analysis. The lysates were also directly probed with the indicated antibodies. ( c ) HisMax-tagged DBC1 and its K-to-R mutants were expressed in HEK293T cells with Flag-SUMO3 and Flag-Ubc9. Cell lysates were treated as in b . In parenthesis, the antibody used for immunoblot analysis of each gel panel was indicated. If not shown, the antibody used was generated directly to the protein indicated by the arrowhead. Note that the membrane blots obtained from immunoprecipitation were typically exposed to X-ray films for about 30 s to show up sumoylated DBC1 bands, while those obtained from cell lysates were for about 2–3 s to show just DBC1 bands for their equal expression. However, sumoylated bands could also be seen in the blots from cell lysates if exposed for a longer period (~30 s). An example is shown in the bottom panel of b full blots in Supplementary Fig. 12 . (See also the bottom panel of Fig. 2a full blots as an additional example). Full size image DNA damage induces DBC1 sumoylation and its binding to SIRT1 Since sumoylation has been implicated in DNA damage response [47] , [48] , we examined whether genotoxic stress induces DBC1 sumoylation. Treatment of U2OS cells with etoposide led to a dramatic increase in SUMO2/3-modification of endogenous DBC1 ( Fig. 2a ). In contrast, little or no SUMO1-conjugated DBC1 could be detected. Similar results were obtained when HeLa cells were treated with doxorubicin ( Supplementary Fig. 1a ). Moreover, knockdown of SUMO2/3 by a SUMO2/3-specific shRNA (shSUMO2/3), but not by a nonspecific shRNA, abrogated etoposide-induced DBC1 sumoylation ( Fig. 2b ), indicating that DBC1 serves as a target for modification by SUMO2/3 under genotoxic stress. 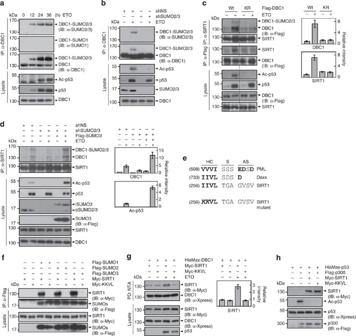Figure 2: Etoposide-induced sumoylation of DBC1 and its interaction with SIRT1. (a) U2OS cells were treated with 20 μM etoposide (ETO) for increasing periods. Their lysates were subjected to immunoprecipitation (IP) with anti-DBC1 antibody followed by immunoblot analysis. Cell lysates were also directly probed with anti-acetylated p53 (Ac-p53), anti-p53 and anti-DBC1 antibodies. (b) U2OS cells expressing nonspecific shRNA (shNS) or shSUMO2/3 were incubated with and without etoposide for 36 h. Their lysates were then treated as ina. (c) HeLa cells expressing Flag-tagged DBC1 (Wt) and its K591R mutant (KR) were incubated with and without etoposide for 36 h. Their lysates were subjected to immunoprecipitation with anti-SIRT1 and anti-Flag antibodies followed by immunoblot analysis (left). The band intensities of DBC1 and SIRT1 obtained from immunoprecipitation were quantified, and those seen by expressing wild-type DBC1 in the absence of etoposide were expressed as 1.0 and the others were expressed as its relative values (right). Error bar, ±s.d. (n=3). (d) HeLa cells expressing shNS or shSUMO2/3 were incubated for 36 h with and without Flag-SUMO3 in the presence and absence of etoposide. Their lysates were then treated as inc. ‘i’ and ‘e’ denote shRNA insensitive and endogenous, respectively (left). The band intensities of DBC1 from immunoprecipitation and acetylated p53 from lysates were quantified. The intensity of DBC1 seen with shNS only and that of Ac-p53 seen with shNS and etoposide were expressed as 1.0 and the others were as its relative values (right). Error bar, ±s.d. (n=3). (e) The SUMO-interacting motifs (SIMs) of PML and Daxx were compared with a similar sequence in SIRT1. Two Ile residues in the hydrophobic core (HC) sequence of SIRT1 were replaced by two Lys residues—S and AS indicate spacer and acidic stretch sequences, respectively. (f) Flag-tagged SUMO isoforms were expressed in HEK293T cells with Myc-tagged SIRT1 or its KKVL mutant. Cell lysates were subjected to immunoprecipitation with anti-Flag antibody followed by immunoblot analysis. (g) HisMax-DBC1 was expressed in HeLa cells with Myc-tagged SIRT1 or its KKVL mutant, and incubated with and without etoposide for 36 h. Cell lysates were subjected to pull-down with NTA-resins followed by immunoblot analysis (left). The band intensities of SIRT1 from immunoprecipitation were quantified, and that seen by expressing HisMax-DBC1 and Myc-SIRT1 in the absence of etoposide was expressed as 1.0 and the others were expressed as its relative values (right). Error bar, ±s.d. (n=3). (h) HisMax-p53 and Flag-p300 were expressed in HeLa cells with Myc-tagged SIRT1 or its KKVL mutant. Cell lysates were subjected to immunoblot analysis. Figure 2: Etoposide-induced sumoylation of DBC1 and its interaction with SIRT1. ( a ) U2OS cells were treated with 20 μM etoposide (ETO) for increasing periods. Their lysates were subjected to immunoprecipitation (IP) with anti-DBC1 antibody followed by immunoblot analysis. Cell lysates were also directly probed with anti-acetylated p53 (Ac-p53), anti-p53 and anti-DBC1 antibodies. ( b ) U2OS cells expressing nonspecific shRNA (shNS) or shSUMO2/3 were incubated with and without etoposide for 36 h. Their lysates were then treated as in a . ( c ) HeLa cells expressing Flag-tagged DBC1 (Wt) and its K591R mutant (KR) were incubated with and without etoposide for 36 h. Their lysates were subjected to immunoprecipitation with anti-SIRT1 and anti-Flag antibodies followed by immunoblot analysis (left). The band intensities of DBC1 and SIRT1 obtained from immunoprecipitation were quantified, and those seen by expressing wild-type DBC1 in the absence of etoposide were expressed as 1.0 and the others were expressed as its relative values (right). Error bar, ±s.d. ( n =3). ( d ) HeLa cells expressing shNS or shSUMO2/3 were incubated for 36 h with and without Flag-SUMO3 in the presence and absence of etoposide. Their lysates were then treated as in c . ‘i’ and ‘e’ denote shRNA insensitive and endogenous, respectively (left). The band intensities of DBC1 from immunoprecipitation and acetylated p53 from lysates were quantified. The intensity of DBC1 seen with shNS only and that of Ac-p53 seen with shNS and etoposide were expressed as 1.0 and the others were as its relative values (right). Error bar, ±s.d. ( n =3). ( e ) The SUMO-interacting motifs (SIMs) of PML and Daxx were compared with a similar sequence in SIRT1. Two Ile residues in the hydrophobic core (HC) sequence of SIRT1 were replaced by two Lys residues—S and AS indicate spacer and acidic stretch sequences, respectively. ( f ) Flag-tagged SUMO isoforms were expressed in HEK293T cells with Myc-tagged SIRT1 or its KKVL mutant. Cell lysates were subjected to immunoprecipitation with anti-Flag antibody followed by immunoblot analysis. ( g ) HisMax-DBC1 was expressed in HeLa cells with Myc-tagged SIRT1 or its KKVL mutant, and incubated with and without etoposide for 36 h. Cell lysates were subjected to pull-down with NTA-resins followed by immunoblot analysis (left). The band intensities of SIRT1 from immunoprecipitation were quantified, and that seen by expressing HisMax-DBC1 and Myc-SIRT1 in the absence of etoposide was expressed as 1.0 and the others were expressed as its relative values (right). Error bar, ±s.d. ( n =3). ( h ) HisMax-p53 and Flag-p300 were expressed in HeLa cells with Myc-tagged SIRT1 or its KKVL mutant. Cell lysates were subjected to immunoblot analysis. Full size image Significantly, SUMO2/3 knockdown also prevented etoposide-induced p53 acetylation ( Fig. 2b ), raising a possibility that DBC1 sumoylation promotes the SIRT1–DBC1 interaction and in turn inhibits SIRT1-mediated deacetylation of p53. To test this possibility, we compared the abilities of DBC1 and its K591R mutant in the interaction with SIRT1. Etoposide treatment led to a dramatic increase in the interaction of SIRT1 with DBC1, but not with the K591R mutant ( Fig. 2c ). Furthermore, knockdown of SUMO2/3 also led to a marked decrease in the DBC1–SIRT1 interaction as well as in p53 acetylation and this decrease could be reversed by complementation of shRNA-insensitive SUMO3 ( Fig. 2d ). Similar results were obtained when the K591R mutant or shSUMO2/3 was expressed in HeLa cells in the presence and absence of doxorubicin ( Supplementary Fig. 1b,c ). We next examined whether the sumoylation-mediated increase in the DBC1–SIRT1 interaction can indeed inhibit the deacetylase activity of SIRT1. Overexpression of SUMO2 or SUMO3, but not SUMO1, with Ubc9 led to a marked increase in the ability of DBC1 to inhibit the SIRT1 activity ( Supplementary Fig. 2a ). Under the same conditions, however, the NAD + /NADH ratio remained unchanged, indicating that the inhibition of the SIRT1 activity is not due to the availability of the SIRT1 substrate ( Supplementary Fig. 2b ). These results indicate that sumoylation of DBC1 is required for its interaction with and inhibition of SIRT1 and in turn for promotion of p53 acetylation under genotoxic stress. SIRT1 has a SIM-like sequence for binding to sumoylated DBC1 In an attempt to determine the mechanical basis for the preferential interaction of SIRT1 with sumoylated DBC1 over its unmodified form, we examined whether SIRT1 has a SUMO-interacting motif (SIM), which consists of hydrophobic core and acidic stretch sequence franked by a spacer [49] , [50] . Sequence analysis showed that SIRT1 has a hydrophobic core sequence (IIVL), which is identical to that of Daxx, although it lacks an acidic stretch ( Fig. 2e ). To determine whether the hydrophobic sequence is involved in the binding of SIRT1 to SUMO, we generated a SIRT1 mutant (KKVL), of which the first two Ile residues were replaced by Lys residues. SIRT1 bound to all of the SUMO isoforms, but this binding could be prevented by the II-to-KK mutation ( Fig. 2f ), indicating that the hydrophobic core of SIRT1 is sufficient for interaction with SUMOs. In addition, purified SUMO3 could effectively compete with SUMO3-conjugated DBC1 for binding to SIRT1 ( Supplementary Fig. 3 ). Furthermore, the II-to-KK mutation prevented the etoposide-mediated increase in the SIRT1–DBC1 interaction ( Fig. 2g ). However, the II-to-KK mutation showed little or no effect on the ability of SIRT1 to deacetylate p53 ( Fig. 2h ), indicating that the effect of the mutation on the SIRT1–DBC1 interaction is not mediated by misfolding or conformational change of SIRT1. These results demonstrate that the SIM-like sequence in SIRT1 is responsible for its interaction with sumoylated DBC1. DBC1 sumoylation blocks the SIRT1–p53 interaction To determine whether DBC1 sumoylation influences the interaction between SIRT1 and p53, HeLa cells overexpressing DBC1 and its K591R mutant were treated with etoposide. Overexpression of DBC1, but not its K591R mutant, markedly decreased the SIRT1–p53 interaction ( Fig. 3a ). Moreover, knockdown of SUMO2/3 led to an increase in the SIRT1–p53 interaction ( Fig. 3b ). Since SUMO2/3 knockdown reduced the DBC1–SIRT1 interaction (see Fig. 2d ), it appeared that sumoylated DBC1, unlike its unmodified form, is capable of replacing p53 for its binding to SIRT1. To test this possibility, increasing amounts of SUMO3 were expressed with a fixed amount of DBC1 or its K591R mutant. The interaction of SIRT1 with DBC1 gradually increased, whereas that with p53 declined in a SUMO3 dose-dependent manner ( Fig. 3c ). In contrast, SIRT1 was unable to interact with the K591R mutant, and remained bound to p53 regardless of SUMO3 expression. These results indicate that sumoylation of DBC1 displaces p53 from SIRT1 for its binding to the deacetylase. 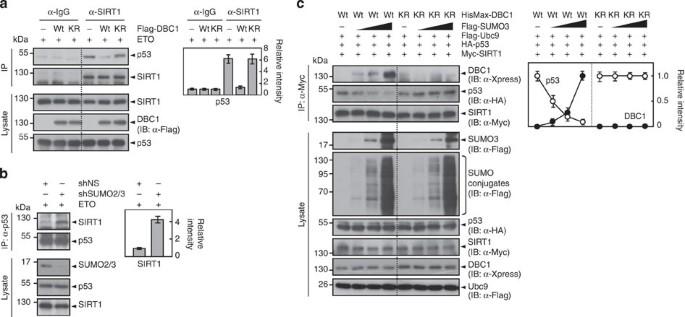Figure 3: DBC1 sumoylation blocks the interaction of SIRT1 with p53. (a) HeLa cells expressing Flag-tagged DBC1 (Wt) or its K591R mutant (KR) were incubated with etoposide for 36 h. Their lysates were subjected to immunoprecipitation with pre-immune IgG or anti-SIRT1 antibody followed by immunoblot analysis (left). The band intensities of p53 from immunoprecipitation were quantified, and that seen without Flag-DBC1 (the first lane) was expressed as 1.0 and the others were expressed as its relative values (right). Error bar, ±s.d. (n=3). (b) HeLa cells expressing nonspecific shRNA (shNS) or shSUMO2/3 were incubated with etoposide for 36 h. Their lysates were subjected to immunoprecipitation with anti-p53 antibody followed by immunoblot analysis (left). The band intensities of SIRT1 from immunoprecipitation were quantified, and that seen with shNS was expressed as 1.0 and the others were expressed as its relative values (right). Error bar, ±s.d. (n=3). (c) HisMax-tagged DBC1 or its K591R mutant, Flag-Ubc9, HA-p53 and Myc-SIRT1 were expressed in HEK293T cells with increasing amounts of Flag-SUMO3. Cell lysates were subjected to immunoprecipitation with anti-Myc antibody followed by immunoblot analysis (left). The band intensities of DBC1 ([cirf ]) and p53 (○) from immunoprecipitation were quantified, and those seen without Flag-SUMO3 were expressed as 1.0 and the others were expressed as its relative values (right). Error bar, ±s.d. (n=3). Figure 3: DBC1 sumoylation blocks the interaction of SIRT1 with p53. ( a ) HeLa cells expressing Flag-tagged DBC1 (Wt) or its K591R mutant (KR) were incubated with etoposide for 36 h. Their lysates were subjected to immunoprecipitation with pre-immune IgG or anti-SIRT1 antibody followed by immunoblot analysis (left). The band intensities of p53 from immunoprecipitation were quantified, and that seen without Flag-DBC1 (the first lane) was expressed as 1.0 and the others were expressed as its relative values (right). Error bar, ±s.d. ( n =3). ( b ) HeLa cells expressing nonspecific shRNA (shNS) or shSUMO2/3 were incubated with etoposide for 36 h. Their lysates were subjected to immunoprecipitation with anti-p53 antibody followed by immunoblot analysis (left). The band intensities of SIRT1 from immunoprecipitation were quantified, and that seen with shNS was expressed as 1.0 and the others were expressed as its relative values (right). Error bar, ±s.d. ( n =3). ( c ) HisMax-tagged DBC1 or its K591R mutant, Flag-Ubc9, HA-p53 and Myc-SIRT1 were expressed in HEK293T cells with increasing amounts of Flag-SUMO3. Cell lysates were subjected to immunoprecipitation with anti-Myc antibody followed by immunoblot analysis (left). The band intensities of DBC1 ([cirf ]) and p53 ( ○ ) from immunoprecipitation were quantified, and those seen without Flag-SUMO3 were expressed as 1.0 and the others were expressed as its relative values (right). Error bar, ±s.d. ( n =3). Full size image PIAS3 serves as a SUMO E3 ligase of DBC1 To identify DBC1-specific SUMO E3 ligase, each of PIAS1-4 was overexpressed with DBC1. Among them, only PIAS3 interacted with DBC1 ( Fig. 4a ). Moreover, the DBC1–PIAS3 interaction was markedly increased by etoposide treatment ( Fig. 4b ). We next examined whether PIAS3 is indeed capable of promoting DBC1 sumoylation. Overexpression of PIAS3 dramatically increased DBC1 sumoylation ( Fig. 4c ). On the other hand, knockdown of PIAS3 by shPIAS3 prevented sumoylation of endogenous DBC1 with a marked reduction in etoposide-induced SIRT1–DBC1 interaction as well as in p53 acetylation ( Fig. 4d ). These effects of PIAS3 knockdown was confirmed by reciprocal immunoprecipitation analysis ( Fig. 4e ). Moreover, complementation of shRNA-insensitive PIAS3 reversed the effects of PIAS3 depletion on both the DBC1–SIRT1 interaction and p53 acetylation, indicating that PIAS3 serves as a SUMO2/3 E3 ligase for DBC1 and in turn as a positive regulator of p53. Of note, however, was the observation that among the proteins immunoprecipitated by anti-SIRT1 antibody ( Fig. 4e ; see also Fig. 2c ), the amount of unmodified DBC1 is significantly higher than that of sumoylated DBC1. Possibly, a portion of SUMO2/3-conjugated DBC1 might have been desumoylated during cell lysate preparation and immunoprecipitation process, although NEM, an inhibitor of desumoylating enzymes were treated in cell lysis buffer. 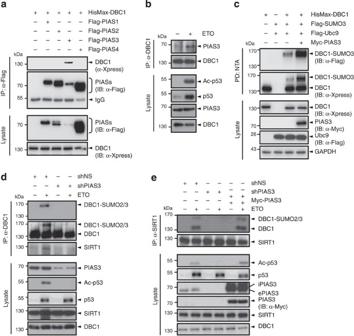Figure 4: PIAS3 serves as a SUMO E3 ligase of DBC1. (a) HisMax-DBC1 was expressed in HEK293T cells with each of Flag-tagged PIAS1-4. Cell lysates were subjected to immunoprecipitation with anti-Flag antibody followed by immunoblot analysis. (b) HeLa cells incubated with and without etoposide for 36 h were subjected to immunoprecipitation with anti-DBC1 antibody followed by immunoblot analysis (left). (c) Flag-tagged SUMO3 and Ubc9 were expressed in HEK293T cells with HisMax-DBC1 and/or Myc-PIAS3. Cell lysates were subjected to pull-down with NTA-resins followed by immunoblot analysis. (d) HeLa cells expressing nonspecific shRNA (shNS) or shPIAS3 were incubated with and without etoposide for 36 h. Their lysates were then treated as inb. (e) shNS and shPIAS3 were expressed in HeLa cells with and without Myc-PIAS3. After incubation with and without etoposide for 36 h, cell lysates were subjected to immunoprecipitation with anti-SIRT1 antibody followed by immunoblot analysis. ‘i’ and ‘e’ denote shRNA insensitive and endogenous, respectively (left). Figure 4: PIAS3 serves as a SUMO E3 ligase of DBC1. ( a ) HisMax-DBC1 was expressed in HEK293T cells with each of Flag-tagged PIAS1-4. Cell lysates were subjected to immunoprecipitation with anti-Flag antibody followed by immunoblot analysis. ( b ) HeLa cells incubated with and without etoposide for 36 h were subjected to immunoprecipitation with anti-DBC1 antibody followed by immunoblot analysis (left). ( c ) Flag-tagged SUMO3 and Ubc9 were expressed in HEK293T cells with HisMax-DBC1 and/or Myc-PIAS3. Cell lysates were subjected to pull-down with NTA-resins followed by immunoblot analysis. ( d ) HeLa cells expressing nonspecific shRNA (shNS) or shPIAS3 were incubated with and without etoposide for 36 h. Their lysates were then treated as in b . ( e ) shNS and shPIAS3 were expressed in HeLa cells with and without Myc-PIAS3. After incubation with and without etoposide for 36 h, cell lysates were subjected to immunoprecipitation with anti-SIRT1 antibody followed by immunoblot analysis. ‘i’ and ‘e’ denote shRNA insensitive and endogenous, respectively (left). Full size image To map the regions for the PIAS3–DBC1 interaction, their deletions were generated ( Supplementary Fig. 4 ). DBC1 bound to the N-terminal region of PIAS3 (amino acids 1–200), and PIAS3 bound to the N-terminal region of DBC1 (1–243). In addition, the deletion of the leucine zipper motif (243–264), which is known to mediate the binding of DBC1 to SIRT1 (ref. 19 ), showed little or no effect on its binding to PIAS3. SENP1 serves as a desumoylating enzyme for DBC1 To identify DBC1-specific desumoylating enzyme, each of SENP1-3 and SENP5-7 was overexpressed with DBC1. Note that SENP4, also called SUSP1, is expressed in rat and mice but not in human [38] . Among the human SENPs, SENP1, SENP3 and SENP5 interacted with DBC1 ( Fig. 5a ). Without overexpression, however, only SENP1 interacted with DBC1 and this interaction was markedly reduced by etoposide treatment ( Fig. 5b ). Since both DBC1 and SENP1 are known to reside in the nucleus [20] , [51] , we examined whether the reduced ability of SENP1 to interact with DBC1 might be due to the change in the locality of SENP1 or DBC1 upon etoposide treatment. Immunocytochemical analysis revealed that endogenous SENP1 and DBC1 proteins co-localize in the nucleus whether treated with etoposide or not ( Supplementary Fig. 5 ), indicating that etoposide-mediated decrease in the SENP1–DBC1 interaction is due to certain reason(s) other than the change in subcellular locality of either protein (see below). 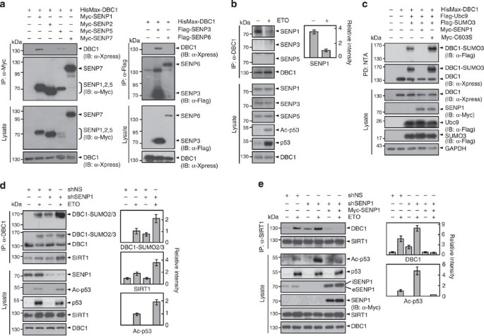Figure 5: SENP1 serves as a desumoylating enzyme for DBC1. (a) HisMax-DBC1 was expressed in HEK293T cells with each of SENP1, 2, 5 and 7 (left) or SENP3 and 6 (right). Cell lysates were subjected to immunoprecipitation with anti-Myc (left) and anti-Flag antibodies (right) followed by immunoblot analysis. (b) HeLa cells incubated with and without etoposide for 36 h were subjected to immunoprecipitation with anti-DBC1 antibody followed by immunoblot analysis (left). The band intensities of SENP1 from immunoprecipitation were quantified, and that seen without etoposide was expressed as 1.0 and the others were expressed as its relative values (right). Error bar, ±s.d. (n=3). (c) HisMax-DBC1, Flag-Ubc9 and Flag-SUMO3 were expressed in HEK293T cells with Myc-tagged SENP1 or its C603S mutant. Cell lysates were subjected to pull-down with NTA-resins followed by immunoblot analysis. (d) HeLa cells expressing nonspecific shRNA (shNS) or shSENP1 were incubated with and without etoposide for 36 h. Their lysates were then treated as inb(left). The band intensities of DBC1-SUMO2/3 (top) and SIRT1 from immunoprecipitation and acetylated p53 from lysates were quantified. The intensities of DBC1-SUMO2/3 and acetylated p53 seen with both shNS and etoposide and that of SIRT1 seen with shNS alone were expressed as 1.0 and the others were expressed as its relative values (right). Error bar, ±s.d. (n=3). (e) shNS and shSENP1 were expressed in HeLa cells with and without Myc-SENP1. They were incubated with and without etoposide for 36 h. Cell lysates were subjected to immunoprecipitation with anti-SIRT1 antibody followed by immunoblot analysis. ‘i’ and ‘e’ denote shRNA insensitive and endogenous, respectively (left). The band intensities of DBC1 from immunoprecipitation and acetylated p53 from lysates were quantified. The intensity of DBC1 seen with shNS only and that of acetylaed-p53 seen with shNS and etoposide were expressed as 1.0 and the others were expressed as its relative values (right). Error bar, ±s.d. (n=3). Figure 5: SENP1 serves as a desumoylating enzyme for DBC1. ( a ) HisMax-DBC1 was expressed in HEK293T cells with each of SENP1, 2, 5 and 7 (left) or SENP3 and 6 (right). Cell lysates were subjected to immunoprecipitation with anti-Myc (left) and anti-Flag antibodies (right) followed by immunoblot analysis. ( b ) HeLa cells incubated with and without etoposide for 36 h were subjected to immunoprecipitation with anti-DBC1 antibody followed by immunoblot analysis (left). The band intensities of SENP1 from immunoprecipitation were quantified, and that seen without etoposide was expressed as 1.0 and the others were expressed as its relative values (right). Error bar, ±s.d. ( n =3). ( c ) HisMax-DBC1, Flag-Ubc9 and Flag-SUMO3 were expressed in HEK293T cells with Myc-tagged SENP1 or its C603S mutant. Cell lysates were subjected to pull-down with NTA-resins followed by immunoblot analysis. ( d ) HeLa cells expressing nonspecific shRNA (shNS) or shSENP1 were incubated with and without etoposide for 36 h. Their lysates were then treated as in b (left). The band intensities of DBC1-SUMO2/3 (top) and SIRT1 from immunoprecipitation and acetylated p53 from lysates were quantified. The intensities of DBC1-SUMO2/3 and acetylated p53 seen with both shNS and etoposide and that of SIRT1 seen with shNS alone were expressed as 1.0 and the others were expressed as its relative values (right). Error bar, ±s.d. ( n =3). ( e ) shNS and shSENP1 were expressed in HeLa cells with and without Myc-SENP1. They were incubated with and without etoposide for 36 h. Cell lysates were subjected to immunoprecipitation with anti-SIRT1 antibody followed by immunoblot analysis. ‘i’ and ‘e’ denote shRNA insensitive and endogenous, respectively (left). The band intensities of DBC1 from immunoprecipitation and acetylated p53 from lysates were quantified. The intensity of DBC1 seen with shNS only and that of acetylaed-p53 seen with shNS and etoposide were expressed as 1.0 and the others were expressed as its relative values (right). Error bar, ±s.d. ( n =3). Full size image To determine whether SENP1 is indeed capable of desumoylating DBC1, we generated a catalytically inactive mutant of SENP1 (C603S) by substituting the active site Cys603 residue by Ser. Overexpression of SENP1, but not its C603S mutant, led to complete desumoylation of DBC1 ( Fig. 5c ). On the other hand, SENP1 knockdown caused a marked increase in DBC1 sumoylation even in the absence of etoposide and this increase was further ameliorated in its presence ( Fig. 5d ). SENP1 knockdown also led to an increase in the DBC1–SIRT1 interaction as well as in p53 acetylation and this increase was further elevated by etoposide treatment. These effects of SENP1 depletion were confirmed by reciprocal immunoprecipitation analysis ( Fig. 5e ). Moreover, complementation of shRNA-insensitive SENP1 reversed the effects of SENP1 depletion on both the DBC1–SIRT1 interaction and p53 acetylation. These results indicate that SENP1 serves as a desumoylating enzyme for DBC1 and in turn as a negative regulator of p53. To map the regions for the SENP1–DBC1 interaction, their deletions were generated. DBC1 bound to the N-terminal region of SENP1 (amino acids 1–200) ( Supplementary Fig. 6a ). Significantly, SENP1 bound to the N-terminal region of DBC1 (1–243) ( Supplementary Fig. 6b ), where PIAS3 also binds (see Supplementary Fig. 4b ). Consistently, SENP1 and PIAS3 were found to compete with each other for binding to DBC1 upon analysis by expression of increasing amounts of the one over the other ( Supplementary Fig. 6c ). These results indicate that DBC1 sumoylation could be dynamically regulated by competitive binding of PIAS3 and SENP1 to DBC1 under genotoxic stress. DBC1 phosphorylation promotes its sumoylation ATM/ATR-mediated phosphorylation of Thr454 in DBC1 was shown to increase its interaction with SIRT1 (refs 25 , 26 ). To determine whether the phosphorylation of DBC1 influences its sumoylation, phosphorylation-defective (T454A) and phosphorylation-mimicking (T454D) mutants were generated by substituting Thr454 with Ala and Asp, respectively. Overexpression of the T454D mutant dramatically increased DBC1 sumoylation, whereas that of the T454A mutant decreased it ( Fig. 6a ). Moreover, the T454D mutation increased the ability of sumoylated DBC1 to bind SIRT1, whereas the T454A mutation decreased it. Furthermore, the T454D mutation promoted the DBC1–PIAS3 interaction, whereas the T454A mutation inhibited it ( Fig. 6b ). In contrast, the T454D mutation decreased the DBC1–SENP1 interaction, whereas the T454A mutation increased it. Consistently, treatment with caffeine, an ATM/ATR inhibitor, prevented the etoposide-induced association and dissociation of DBC1 with PIAS3 and SENP1, respectively ( Fig. 6c ). These results indicate that ATM/ATR-mediated DBC1 phosphorylation serves as a switch of DBC1-binding partner from SENP1 to PIAS3 for DBC1 sumoylation, which in turn promotes the DBC1–SIRT1 interaction for p53 acetylation under genotoxic stress. 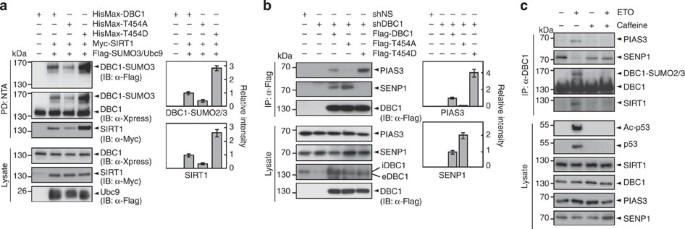Figure 6: DBC1 phosphorylation promotes its sumoylation. (a) Flag-tagged SUMO3 and Ubc9 were expressed in HEK293T cells with HisMax-tagged DBC1, T454A or T454D. Cell lysates were subjected to pull-down with NTA-resins followed by immunoblot analysis (left). The band intensities of DBC1-SUMO3 (top) and SIRT1 from immunoprecipitation were quantified, and those seen with HisMax-DBC1, Myc-SIRT1 and Flag-tagged SUMO3 and Ubc9 were expressed as 1.0 and the others were expressed as its relative values (right). Error bar, ±s.d. (n=3). (b) shRNA-insensitive Flag-tagged DBC1, T454A or T454D was expressed in HeLa cells that had been stably transfected with nonspecific shRNA (shNS) or shDBC1. Cell lysates were subjected to immunoprecipitation with anti-Flag antibody followed by immunoblot analysis (left). The band intensities of PIAS3 and SENP1 from immunoprecipitation were quantified, and those seen with both shDBC1 and Flag-DBC1 were expressed as 1.0 and the others were expressed as its relative values (right). Error bar, ±s.d. (n=3). (c) HeLa cells were incubated with etoposide and/or 5 mM caffeine for 36 h. Cell lysates were subjected to immunoprecipitation with anti-DBC1 antibody followed by immunoblot analysis. Figure 6: DBC1 phosphorylation promotes its sumoylation. ( a ) Flag-tagged SUMO3 and Ubc9 were expressed in HEK293T cells with HisMax-tagged DBC1, T454A or T454D. Cell lysates were subjected to pull-down with NTA-resins followed by immunoblot analysis (left). The band intensities of DBC1-SUMO3 (top) and SIRT1 from immunoprecipitation were quantified, and those seen with HisMax-DBC1, Myc-SIRT1 and Flag-tagged SUMO3 and Ubc9 were expressed as 1.0 and the others were expressed as its relative values (right). Error bar, ±s.d. ( n =3). ( b ) shRNA-insensitive Flag-tagged DBC1, T454A or T454D was expressed in HeLa cells that had been stably transfected with nonspecific shRNA (shNS) or shDBC1. Cell lysates were subjected to immunoprecipitation with anti-Flag antibody followed by immunoblot analysis (left). The band intensities of PIAS3 and SENP1 from immunoprecipitation were quantified, and those seen with both shDBC1 and Flag-DBC1 were expressed as 1.0 and the others were expressed as its relative values (right). Error bar, ±s.d. ( n =3). ( c ) HeLa cells were incubated with etoposide and/or 5 mM caffeine for 36 h. Cell lysates were subjected to immunoprecipitation with anti-DBC1 antibody followed by immunoblot analysis. Full size image DBC1 sumoylation is required for p53 transactivation To determine whether DBC1 sumoylation leads to transcriptional activation of p53 by sequestering SIRT1 from p53, two reporter vectors, PG13-LUC and BAX-LUC , were employed. Etoposide treatment increased in the luciferase activity and this increase was further elevated by overexpression of DBC1, but not by that of the K591R mutant ( Fig. 7a ). Moreover, knockdown of SUMO2/3 or PIAS3 abrogated etoposide-induced p53 transactivity regardless of co-knockdown of DBC1 ( Fig. 7b ). In contrast, knockdown of SENP1 further increased the drug-induced p53 transactivity and this increase was abrogated by co-knockdown of DBC1 ( Fig. 7c ). Cells used for Fig. 7a–c were subjected to immunoblot analysis to confirm the overexpression or knockdown of the indicated proteins ( Fig. 7d–f , respectively). These results indicate that DBC1 sumoylation is required for transcriptional activation of p53 under genotoxic stress. 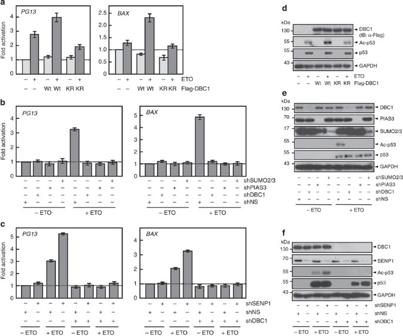Figure 7: DBC1 sumoylation is required for p53 transactivation. (a) Flag-DBC1 (Wt) or its K591R mutant (KR) was expressed in HeLa cells withPG13-Luc(left) orBAX-Luc(right). After incubation with and without etoposide for 36 h, cells were subjected to assay for the luciferase activity. The activity seen without any treatment was expressed as 1.0 and the others were expressed as its relative values. (b) Nonspecific shRNA (shNS), shDBC1, shPIAS3 or shSUMO2/3 was expressed in HeLa cells withPG13-Luc(left) orBAX-Luc(right). They were then treated as ina. (c) shNS or shDBC1 and/or shSENP1 was expressed in HeLa cells withPG13-Luc(left) orBAX-Luc(right). They were then treated as ina. Error bar, ±s.d. (n=3). (d–f) Cells prepared, as ina–c, were subjected to immunoblot analysis. Figure 7: DBC1 sumoylation is required for p53 transactivation. ( a ) Flag-DBC1 (Wt) or its K591R mutant (KR) was expressed in HeLa cells with PG13-Luc (left) or BAX-Luc (right). After incubation with and without etoposide for 36 h, cells were subjected to assay for the luciferase activity. The activity seen without any treatment was expressed as 1.0 and the others were expressed as its relative values. ( b ) Nonspecific shRNA (shNS), shDBC1, shPIAS3 or shSUMO2/3 was expressed in HeLa cells with PG13-Luc (left) or BAX-Luc (right). They were then treated as in a . ( c ) shNS or shDBC1 and/or shSENP1 was expressed in HeLa cells with PG13-Luc (left) or BAX-Luc (right). They were then treated as in a . Error bar, ±s.d. ( n =3). ( d – f ) Cells prepared, as in a – c , were subjected to immunoblot analysis. Full size image DBC1 sumoylation is required for p53-mediated apoptosis To determine whether DBC1 sumoylation-mediated p53 activation is responsible for DNA damage-induced apoptosis, we generated HeLa cells that stably express nonspecific shRNA or shDBC1. As expected, DBC1 knockdown prevented etoposide-mediated increase in the cleavage of PARP1 and caspase-9 and the level of acetylated p53 ( Fig. 8a ). However, complementation of shRNA-insensitive DBC1, but not the K591 mutant, led to a significant increase in both of them in the presence of etoposide, but not in its absence. Knockdown of SENP1 also increased the cleavage of PARP1 and caspase-9 and the level of acetylated p53 and this increase could be abrogated by co-knockdown of DBC1 ( Fig. 8b ). On the other hand, knockdown of SUMO2/3 or PIAS3 prevented both of them and these effects could be reversed by co-expression of shRNA-insensitive SUMO3 or PIAS3, respectively ( Fig. 8c ). Consistently, overexpression of DBC1, but not the K591R mutant, markedly increased the number of TUNEL-positive apoptotic cells ( Fig. 8d and Supplementary Fig. 7a ). Whereas knockdown of SUMO2/3 or PIAS3 decreased the number of apoptotic cells, that of SENP1 increased the number and this increase was abrogated by co-knockdown of DBC1 ( Fig. 8e and Supplementary Fig. 7b ). Similar results were obtained when the experiments for Fig. 8a,d were performed in the presence and absence of doxorubicin ( Supplementary Fig. 8a,b , respectively). These results indicate that DBC1 sumoylation is a crucial step for p53-mediated apoptosis under genotoxic stress. 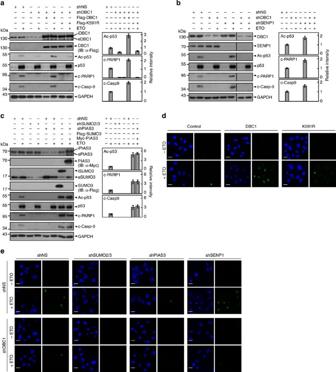Figure 8: DBC1 sumoylation is required for p53-mediated apoptosis. (a) shRNA-insensitive Flag-tagged DBC1 or its K591R mutant was expressed in HeLa cells that had been stably transfected with nonspecific shRNA (shNS) or shDBC1. After incubation with and without etoposide for 36 h, they were subjected to immunoblot with anti-DBC1, anti-acetyl p53, anti-cleaved PARP1 and anti-cleaved caspase-9 (Casp-9) antibodies. ‘c’ denotes cleaved (left). The band intensities of acetylated p53, c-PARP1 and c-Casp-9 from lysates were quantified, and those seen with both shNS and etoposide were expressed as 1.0 and the others were expressed as its relative values (right). Error bar, ±s.d. (n=3). (b) shNS or shDBC1 was expressed in HeLa cells with or without shSENP1. Cells were then incubated in the presence and absence of etoposide for 36 h (left). The band intensities of acetylated p53, c-PARP1 and c-Casp-9 were quantified as ina(right). Error bar, ±s.d. (n=3). (c) shSUMO2/3 or shPIAS3 was expressed in HeLa cells with Flag-SUMO3 or Myc-PIAS3 (left). The band intensities were quantified as ina(right). Error bar, ±s.d. (n=3). (d) HeLa cells expressing Flag-DBC1 or its K591R mutant were incubated with and without etoposide for 36 h. They were then subjected to TUNEL assay. Scale bars, 20 μm. (e) shNS or shDBC1 was expressed in HeLa cells with shNS, shSUMO2/3, shPIAS3 or shSENP1. After incubation with and without etoposide, cells were subjected to TUNEL assay. Ina,c, ‘i’ and ‘e’ denote shRNA insensitive and endogenous, respectively. Scale bars, 20 μm. Figure 8: DBC1 sumoylation is required for p53-mediated apoptosis. ( a ) shRNA-insensitive Flag-tagged DBC1 or its K591R mutant was expressed in HeLa cells that had been stably transfected with nonspecific shRNA (shNS) or shDBC1. After incubation with and without etoposide for 36 h, they were subjected to immunoblot with anti-DBC1, anti-acetyl p53, anti-cleaved PARP1 and anti-cleaved caspase-9 (Casp-9) antibodies. ‘c’ denotes cleaved (left). The band intensities of acetylated p53, c-PARP1 and c-Casp-9 from lysates were quantified, and those seen with both shNS and etoposide were expressed as 1.0 and the others were expressed as its relative values (right). Error bar, ±s.d. ( n =3). ( b ) shNS or shDBC1 was expressed in HeLa cells with or without shSENP1. Cells were then incubated in the presence and absence of etoposide for 36 h (left). The band intensities of acetylated p53, c-PARP1 and c-Casp-9 were quantified as in a (right). Error bar, ±s.d. ( n =3). ( c ) shSUMO2/3 or shPIAS3 was expressed in HeLa cells with Flag-SUMO3 or Myc-PIAS3 (left). The band intensities were quantified as in a (right). Error bar, ±s.d. ( n =3). ( d ) HeLa cells expressing Flag-DBC1 or its K591R mutant were incubated with and without etoposide for 36 h. They were then subjected to TUNEL assay. Scale bars, 20 μm. ( e ) shNS or shDBC1 was expressed in HeLa cells with shNS, shSUMO2/3, shPIAS3 or shSENP1. After incubation with and without etoposide, cells were subjected to TUNEL assay. In a , c , ‘i’ and ‘e’ denote shRNA insensitive and endogenous, respectively. Scale bars, 20 μm. Full size image We next examined whether the removal of etoposide from media could reverse the drug-induced DBC1 sumoylation and apoptosis. Withdrawal of etoposide from culture media at 48 h led to a sharp decrease in the levels of sumoylated DBC1, p53 and acetylated p53 ( Supplementary Fig. 9 ). On the other hand, the levels of cleaved PARP1 and caspase-9 remained elevated, although did not increase any further. These results indicate that the damaged cells could not escape from apoptosis even after the removal of etoposide. It has been shown that SIRT1 localized in the cytoplasm can enhance apoptosis independently of its deacetylase activity, but dependently on caspases [52] , [53] . Therefore, we examined whether etoposide might induce the cytoplasmic localization of SIRT1. Immunocytochemical analysis revealed that the drug treatment rather slightly increases the nuclear localization of both endogenous and ectopically expressed SIRT1 proteins ( Supplementary Fig. 10a ). In addition, etoposide-mediated increase in the cleavage of PARP1 and caspase-9 and the level of acetylated p53 could be prevented by overexpression of SIRT1, but not by that of its catalytically inactive SIRT1 (H363Y), of which the active site His363 residue was replaced by Tyr ( Supplementary Fig. 10b ), confirming that the enzyme activity of SIRT1 is involved in negative regulation of p53-mediated apoptosis. Based on the present findings, we propose a model for the role of DBC1 sumoylation in the control of p53-mediated apoptosis in response to DNA damage ( Supplementary Fig. 11 ). DBC1 is normally bound to SENP1. Under genotoxic stress, however, DBC1 becomes phosphorylated at Thr454 by the ATM/ATR kinases [25] , [26] and this phosphorylation switches the binding partner of DBC1 from SENP1 to PIAS3, leading to its sumoylation. DBC1 sumoylation markedly increases the DBC1–SIRT1 interaction and this tight binding displaces p53 from SIRT1, allowing acetylation (for example, by p300) and transactivation of p53 for the expression of its downstream genes, such as BAX and PUMA, which induce apoptotic cell death. Interestingly, DBC1 was modified by SUMO2/3, but not by SUMO1, despite the fact that PIAS3 is capable of modifying other target proteins by SUMO1, such as hnRNP-K [47] . Moreover, SIRT1 has a SIM-like sequence, which can bind SUMO2/3, suggesting that SUMO2/3 conjugated to DBC1 increases the affinity of the inhibitor protein to SIRT1. Collectively, post-translational modifications of DBC1 by the sequential actions of ATM/ATR kinases and PIAS3 play a crucial role in the control of the DBC1–SIRT1 interaction for p53-mediated apoptosis under genotoxic stress. SUMO2/3, unlike SUMO1, is known to form poly-SUMO chains. However, DBC1 was found to be modified by a single molecule of SUMO2/3 (mono-SUMO2/3-ylated), but not by its polymeric chain. Likewise, Drp1 and RORα have been shown to be mono-SUMO2/3-ylated [54] , [55] . Thus, it seems likely that SUMO2/3 can be conjugated to target proteins not only as polymeric chain(s) but also as a single molecule, although it remains unknown how the chain length is regulated. Of interest was the finding that SENP1 and PIAS3 bind to the same N-terminal region of DBC1 and this competitive binding can be switched by ATM/ATR-mediated phosphorylation of DBC1. However, it remains unknown how the phosphorylation of DBC1 at Thr454, which is located distal to the binding region (the amino acids 1–243) of SENP1 and PIAS3, could influence the interaction of DBC1 with the SUMO-modifying enzymes. Possibly in the three-dimensional structure of DBC1, Thr454 may be in close proximity to the binding site for SENP1 and PIAS3, and when the Thr residue is phosphorylated, the negative charge might provide a better structural atmosphere for the interaction of DBC1 with PIAS3, but not with SENP1. Recently, it has been reported that ATM-mediated phosphorylation of DBC1 at Thr454 provides a second binding site for SIRT1, leading to inhibition of the deacetylase activity [25] . Notably, DBC1 is capable of forming a ternary complex with PIAS3 and SIRT1 upon treatment with etoposide and this complex formation could be prevented by co-treatment with caffeine, an inhibitor of the ATM/ATR kinases ( Fig. 6c ). Thus, it appears possible that DBC1 phosphorylation plays a dual role: one in providing a second binding site for SIRT1 and the other in promotion of PIAS3 binding to DBC1 for sumoylation, which further increases the DBC1–SIRT1 interaction via the SIM-like sequence of the deacetylase. Significantly, SIRT1 can be modified by SUMO1 and this modification increases its deacetylase activity, leading to p53 inactivation and cell survival [15] . Under stress conditions, however, SENP1 inactivates SIRT1 by desumoylation and in turn activates p53 for stress-induced apoptosis. Therefore, SIRT1 sumoylation was suggested to act as a molecular switch that tips the balance from survival to death when DNA is damaged [15] , although it was not determined whether SIRT1 sumoylation influences its ability to interact with DBC1. Interestingly, the same SENP1 enzyme is utilized for desumoylation of both SIRT1 and DBC1, although the enzyme removes SUMO1 from SIRT1 and SUMO2/3 from DBC1. However, SENP1-mediated desumoylation of SIRT1 and DBC1 appears to oppositely impact on cell fate. Whereas the action of SENP1 on SIRT1 promotes stress-induced apoptosis by inactivating the deacetylase activity, its action on DBC1 allows cells to survive by inhibiting the DBC1–SIRT1 interaction under unstressed conditions. DBC1 may sequester SENP1 from SIRT1 under normal conditions ( Fig. 5b ) and thereby SIRT1 would maintain its sumoylated state for p53 deacetylation. However, when DBC1 is phosphorylated in response to DNA damage, SENP1 bound to DBC1 would be replaced by PIAS3 and become available for desumoylation of SIRT1. In conclusion, we demonstrated that the modification of DBC1 by SUMO2/3 orchestrates with its ATM/ATR-mediated phosphorylation and SENP1-mediated removal of SUMO1 from SIRT1 for the control of the DBC1–SIRT1 interaction and in turn for p53-mediated apoptosis under genotoxic stress. Importantly, however, DBC1 has also been implicated in promotion of cell proliferation [56] . For example, DBC1 binds to ERα, but its knockdown in MCF7 breast cancer cells enhances apoptosis in the absence of oestrogen, suggesting the role of DBC1 as a positive regulator of cell growth [57] . Furthermore, it has been shown that the mRNA level of DBC1 is upregulated in breast cancers, although not in prostate cancers [58] , [59] , [60] . Thus, it appears that DBC1 plays a pleiotropic role in the control of cell growth and death, which might depend on cell and tissue types. Plasmids and shRNAs The complementary DNA (cDNA) of DBC1 was cloned into pcDNA-HisMax and pCMV2-Flag. shRNAs were purchased from Open Biosystems. Target sequences for shRNAs are as follows: shPIAS3, 5′-GCTGTCGGTCAGACATCATTT-3′; shSENP1, 5′-CAAAGATATTCAAACTCTA-3′; shSUMO2/3, 5′-TCAATGAGGCAGATCAGATTC-3′. Cell culture and transfection HEK293T, U2OS and HeLa (ATCC: CCL-2) cells were grown at 37 °C in DMEM supplemented with 100U ml −1 penicillin, 1 mg ml −1 streptomycin and 10% foetal bovine serum. All transfections were carried out using Metafectene reagent (Biontex) and jetPEI DNA Transfection Reagent (Polyplus-transfection). Assays for SUMO modification HisMax-DBC1, Flag-SUMO3 and Flag-Ubc9 were overexpressed in HEK293T cells with or without Myc-tagged PIAS3 or SENP1. After culturing for 40 h, cells were lysed by boiling for 10 min in 150 mM Tris-HCl (pH 8), 5% SDS and 30% glycerol. Cell lysates were diluted 20-fold with buffer A (20 mM Tris-HCl (pH 8.0), 150 mM NaCl, 1% Triton X-100, 1 × protease inhibitor cocktail (Roche)) containing 10 mM imidazole and 2 mM NEM. After incubating them with Ni 2+ –NTA–agarose for 2 h at 4 °C, the resins were collected, washed with buffer A containing 20 mM imidazole, and boiled in SDS-sampling buffer. Supernatants were subjected to SDS–polyacrylamide gel electrophoresis (SDS–PAGE) followed by immunoblot analysis. For assaying sumoylation of endogenous DBC1, HeLa cells treated with and without etoposide were lysed as above. Cell lysates were diluted 20-fold with buffer B (20 mM Tris-HCl (pH 8.0), 150 mM NaCl, 0.1 mM EDTA and 1 × protease inhibitor cocktail) containing 0.2% Triton X-100 and 4 mM NEM. The samples were incubated with anti-DBC1 antibody for 2 h at 4 °C and then with protein-A-Sepharose for the next 2 h. The resins were collected, washed with buffer B containing 1% Triton X-100 and boiled. Supernatants were subjected to SDS–PAGE followed by immunoblot analysis. Immunoprecipitation Cell lysates were prepared in buffer B containing 1% Triton X-100 and 2 mM NEM. Cell lysates were incubated with appropriate antibodies for 2 h at 4 °C and then with protein A-conjugated Sepharose for the next 1.5 h. Supernatants were subjected to SDS–PAGE followed by immunoblot analysis. Full scans of immunoblots are presented in Supplementary Fig. 12 . Antibodies against p53 (catalogue#: DO-1), GAPDH (2D4A7), Ubc9 (N-15), DBC1 (H-2) and SENP1 (C-12) were purchased from Santa Cruz. Anti-acetyl p53 (Millipore, 04-1146), anti-DBC1 (Bethyl, A300-434A) and anti-Flag M2 (Sigma-Aldrich, 1804) were also used. Anti-Xpress (1405573), anti-SUMO-1 (381900) and anti-SUMO2/3 (51-9100) were purchased from Invitrogen. Anti-PIAS3 (4164S), anti-cleaved caspase-9 (7237S) and anti-cleaved PARP1 (9541) were purchased from Cell signaling. For immunoblot analysis, all antibodies were diluted 1,000-fold in 3% BSA solution, except anti-Xpress and Flag M2 antibodies, which were diluted 5,000-fold. Quantification of blotted protein bands Protein bands obtained by immunoblot and immunoprecipitation analyses were scanned using a densitometer and their densities were quantified using ‘Image J’ programme. Data were presented as the mean±s.d. of three independent experiments. SIRT1 activity assay The decetylase activity of SIRT1 was determined by using a SIRT1 Activity Assay Kit (Abcam: catalogue# ab156065) as recommended by the manufacturer. Briefly, cells were washed with cold PBS, lysed in buffer B containing 0.2% Triton X-100 and incubated on ice for 5 min. Cell lysates were treated with anti-SIRT1 antibody for 2 h at 4 °C and then with protein A-conjugated Sepharose for the next 1.5 h. Precipitates were incubated with Fluoro-Substrate Peptide Solution, NAD + and SIRT1 Assay Buffer. Fluorescence intensity was then measured using a microtitre plate fluorometer with excitation at 350 nm and emission at 450 nm. Determination of NAD + /NADH ratio Intracellular NAD + /NADH ratio was determined by using the NAD + /NADH Quantification Colorimetric Kit (BioVision: catalogue# K337-100) as recommended by the manufacturer. Briefly, cells were washed with ice-cold PBS and disrupted by freezing-and-thawing. After centrifugation, one half of the extracts were subjected to quantification of the total amount of NAD + plus NADH by using appropriate buffers and reagents provided by the manufacturer. The other half was heated at 60 °C for 30 min to decompose NAD + , followed by determination of the amount of heat-stable NADH. The ratio of NAD + /NADH was then calculated by subtracting the amount of NADH from the total amount of NAD + plus NADH and then divided by the amount of NADH. Purification of SUMO3, sumoylated DBC1 and SIRT1 To obtain free SUMO3 molecules, Flag-SUMO3 was expressed in HEK293T cells. Cell lysates were incubated with anti-Flag-Sepharose (Sigma) for 2 h. The beads were collected, incubated with Flag peptides (Sigma) for 30 min and centrifuged. The supernatants were used as purified SUMO3. To obtain sumoylated DBC1, HisMax-DBC1, Flag-SUMO3 and Myc-Ubc9 were expressed in HEK293T cells. Cell lysates were then treated as above. The proteins eluted from the beads by Flag peptides were incubated with NTA-resins for 2 h. The resins were collected, incubated with PBS containing 200 mM imidazole for 30 min and centrifuged. The supernatants were used as the purified SUMO3-conjugated DBC1. To purify SIRT1, glutatione S-transferase–SIRT1 was expressed in Escherichia coli (BL21). Cell extracts were incubated with glutathione-Sepharose (GE). The beads were collected, incubated with glutathione. The supernatants were used as the purified glutatione S-transferase–SIRT1. All of the protein purifications were carried out at 4 °C. Luciferase assays HeLa cells transfected with pcDNA-β-Gal and PG13-Luc or BAX-Luc were incubated for 48 h. After etoposide treatment, cells were cultured for 30 h, harvested and assayed for luciferase. The enzyme activity was measured in a luminometer and normalized by β-galactosidase expression with a luciferase system (Promega). TUNEL assay After treatment with etoposide, HeLa cells were permeabilized by incubation in a solution containing 0.1% sodium citrate and 0.1% Triton X-100 for 30 min at 65 °C. After extensive washing, samples were further incubated in the Terminal deoxynucleotidyl transferase dUTP Nick End Labelling (TUNEL) reaction solutions of the in situ cell death detection kit (Roche Applied Science) at 37 °C. How to cite this article : Park, J. H. et al. Modification of DBC1 by SUMO2/3 is crucial for p53-mediated apoptosis in response to DNA damage. Nat. Commun. 5:5483 doi: 10.1038/ncomms6483 (2014).